Kinetic inductance magnetometer Sensing ultra-low magnetic fields has various applications in the fields of science, medicine and industry. There is a growing need for a sensor that can be operated in ambient environments where magnetic shielding is limited or magnetic field manipulation is involved. To this end, here we demonstrate a new magnetometer with high sensitivity and wide dynamic range. The device is based on the current nonlinearity of superconducting material stemming from kinetic inductance. A further benefit of our approach is of extreme simplicity: the device is fabricated from a single layer of niobium nitride. Moreover, radio frequency multiplexing techniques can be applied, enabling the simultaneous readout of multiple sensors, for example, in biomagnetic measurements requiring data from large sensor arrays. Ultrasensitive magnetic detection is utilized in a variety of applications, such as magnetoencephalography [1] , magnetocardiography [2] , ultra-low-field NMR [3] and magnetic resonance imaging (ULF NMR and MRI) [4] , [5] , [6] , exploration of magnetic minerals [7] and a wide range of other scientific purposes. The most established method is to use superconducting quantum interference devices (SQUIDs) based on low critical temperature superconducting materials [8] , [9] as the sensor, featuring field sensitivity in the fT Hz −1/2 regime or below. In some applications, their high critical temperature counterparts are an option as well [10] . Emerging sensing techniques include magnetometers combining the giant magnetoresistance effect and a superconducting receiver coil, the mixed sensors [11] and atomic magnetometers relying on the interaction of magnetic field and optically manipulated electronic spins of alkali vapour atoms [12] . Also, the magnetic manipulation of the density of states in normal metal–superconductor interfaces has been proposed, in a so-called superconducting quantum interference proximity transistor [13] . Kinetic inductance of superconductors has been actively pursued in the fields of submillimeter-wave detection [14] , [15] and parametric amplification [16] during the last decade. There have been a few demonstrations of kinetic inductance being used as a sensing element in a magnetic field detector as well. Yet, the reported characteristics have been far inferior in comparison with competing techniques. Meservey and Tedrow [17] were the first ones to observe shifts in kinetic inductance of superconducting thin film under perpendicular magnetic field, detecting a field change of 1 nT. A more advanced magnetic flux detector was proposed [18] , employing a scheme similar to radio frequency (RF) SQUIDs. Instead of having a tunnel junction, a thin superconducting bridge was deposited as a part of superconducting cylinder. The nonlinear relation between the kinetic inductance of the constriction and the magnetic flux applied through the cylinder was read out with a tank circuit. Later, taking advantage of the divergence of the kinetic inductance near critical temperature T c , Ayela et al. [19] applied thermal modulation to a superconducting ring to enhance its field sensitivity down to pT Hz −1/2 . Recently, a set of new nonlinear kinetic inductance devices was proposed by Kher et al. [20] , including a magnetic field sensor. In this article, we demonstrate a magnetometer exploiting the nonlinearity of the kinetic inductance with respect to d.c. current, often encountered in high normal resistance thin films. As opposed to ref. 18 , the entire superconducting loop, having integrated tuning and matching capacitors, acts as a distributed nonlinear element. This improves the sensitivity, enables the use of large pickup sizes and simplifies the design since external tank circuit is not necessary. The device is fabricated from a single superconducting thin-film layer of NbN, simplifying the fabrication processes compared with other magnetometer technologies considerably. In addition, the technology is compatible with frequency-division multiplexing in analogy to submillimeter-wave kinetic inductance detectors [21] , enabling a compact readout of an array of sensors. Large sensor arrays are needed, for instance, in biomagnetic imaging systems relying on inverse mathematics in source mapping [22] . The device performance is evaluated both theoretically and experimentally with the results in good agreement with each other. Operating principle Consider a superonducting loop composed of thin film with thickness h and linewidth w . When h ≪ λ , the current density J s can be assumed to be homogeneous within the cross-section and the magnetic flux quantization through the ring reads where λ is the magnetic penetration depth, I s = J s wh the shielding current, Φ a the applied magnetic flux, m an integer and Φ 0 =2.07 fWb the flux quantum. Unlike the geometric inductance L g that is associated with the magnetic field of the ring, the kinetic inductance L k = μ 0 λ 2 l / wh ( μ 0 is the vacuum permeability and l the length of the loop) stems from the motion of the Cooper pairs. Kinetic inductance becomes nonlinear with respect to shielding current I s as the kinetic energy approaches the depairing energy of the Cooper pairs [16] , [23] . With sufficiently small I s , the nonlinearity assumes a form Here, L k0 is the kinetic inductance at zero current and I *, a parameter usually of the order of critical current I c , sets the scale for the nonlinearity. The operating principle behind the kinetic inductance magnetometer is as follows: the magnetic flux Φ a applied through the loop (inductance L = L g + L k ) generates a shielding current I s according to equation (1), which in turn modifies the inductance of the loop through equation (2). 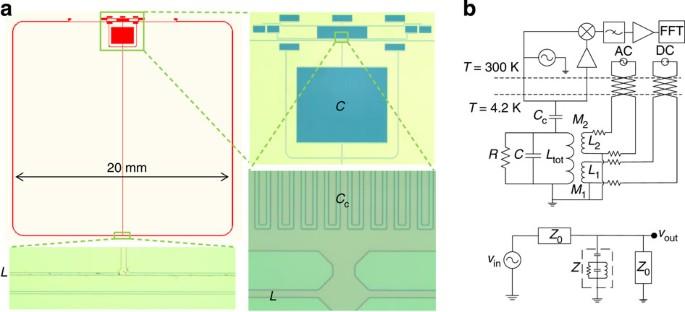Figure 1: Magnetometer design and simplified circuit diagrams for the setup and the transmission measurement. (a) The device contains a superconducting loopLfabricated employing a single NbN thin-film layer. The interdigital capacitorsCandCc, shown in the optical microphotograph zoom-ins, are placed inside and outside the loop, respectively. Together with the inductive loop, the capacitors form a resonator coupled to an external transmission line. A superconducting on-chip bias coil concentric withLwas not employed in the experiments. (b) Two off-chip coilsL1andL2with calibrated mutual inductances (M1andM2) are arranged around the magnetometer loop to generate bias and excitation fluxes. An RF generator supplies excitation and reference signals for the resonator and mixer, respectively. The applied magnetic field changes the kinetic inductance of the loop affecting the transmission spectrum of the microwaves passing the resonator. The resulting signal, being proportional to the excitation voltageεin, is amplified, mixed down to d.c. and finally Fourier transformed to frequency domain. All experiments were performed at liquid helium bath temperatureT=4.2 K. (c) TransmissionS21can be modelled with an equivalent circuit, which yieldsS21=2εout/εin=2Z/(2Z+Z0). Figure 1a shows a practical realization of such a device in planar geometry along with the simplified measurement setup depicted in Fig. 1b . A square-shaped superconducting loop (width W =20 mm) has been fabricated from thin-film NbN ( T c =14 K). An interdigital capacitor C is arranged in parallel with the loop, and the formed resonator is further coupled to a transmission line (characteristic impedance Z 0 =50 Ω) with a matching capacitor C c . After cooling the device below T c , the inductance change is read out by measuring the transmission S 21 =2 Z /(2 Z + Z 0 ) through the resonator, which near the resonance frequency is determined by impedance ( Fig. 1c ) Figure 1: Magnetometer design and simplified circuit diagrams for the setup and the transmission measurement. ( a ) The device contains a superconducting loop L fabricated employing a single NbN thin-film layer. The interdigital capacitors C and C c , shown in the optical microphotograph zoom-ins, are placed inside and outside the loop, respectively. Together with the inductive loop, the capacitors form a resonator coupled to an external transmission line. A superconducting on-chip bias coil concentric with L was not employed in the experiments. ( b ) Two off-chip coils L 1 and L 2 with calibrated mutual inductances ( M 1 and M 2 ) are arranged around the magnetometer loop to generate bias and excitation fluxes. An RF generator supplies excitation and reference signals for the resonator and mixer, respectively. The applied magnetic field changes the kinetic inductance of the loop affecting the transmission spectrum of the microwaves passing the resonator. The resulting signal, being proportional to the excitation voltage ε in , is amplified, mixed down to d.c. and finally Fourier transformed to frequency domain. All experiments were performed at liquid helium bath temperature T =4.2 K. ( c ) Transmission S 21 can be modelled with an equivalent circuit, which yields S 21 =2 ε out / ε in =2 Z /(2 Z + Z 0 ). Full size image assuming Q i >>1. Here, Q i is the intrinsic quality factor describing the superconductor losses, the coupling quality factor and the inductance L tot = L /4+ L par contains the contributions from the loop inductance and parasitics. The resonator impedance reaches a real value Z min ≈ Z 0 Q ext /(2 Q i ) at the resonance, creating a decline in S 21 depicted in Fig. 2a,b . We quantify the magnetic bias and excitation as an average orthogonal field B 0 =Φ a / A with A the surface area of the loop. As the applied field B 0 , and consequently I s (assuming m =0), is adjusted between zero and a maximum value, the resonance dip f 0 = ω 0 /(2 π ) shifts between points O and P, respectively. When I s is driven above I c =10 mA (point P), the integer m assumes a new value and the current I s resets according to equation (1). For most of our devices, I s drops close to zero after exceeding the critical current and the resonance dip hops back from state P to state O. 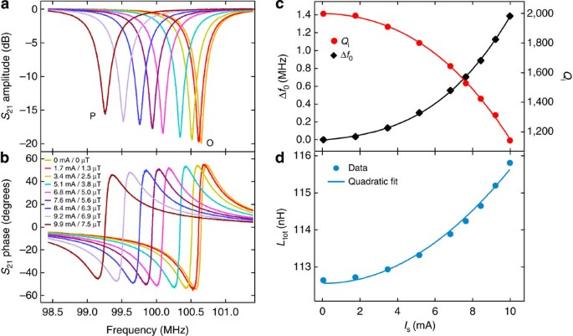Figure 2: Transmission spectra and derived device parameters. (a,b) Resonator transmissionS21was measured with a network analyser as a function of the screening currentIsand bias fieldB0. (c) The intrinsic quality factorof the resonator and the resonance frequency shift Δf0=f0(Is=0)−f0(Is) have been obtained from transmission curves ofa,b(see Methods). Solid lines present polynomial fits. (d) The inductanceLtotdetermines the resonance frequency according to, whereC=20 pF andCc=2.2 pF. The inductanceLtot=(Lg+Lk)/4+Lparcontains contributions from loop inductance and parasitics, whereLg=142 nH andLpar=Lg,par+Lk0,par=40 nH with geometric inductances computed with a simulation software. The quadratic fit ofdgivesLk0=147 nH andI*=34 mA for the kinetic inductance. As the external field is changed further, the resonance frequency f 0 starts again the approach towards point P. Figure 2: Transmission spectra and derived device parameters. ( a , b ) Resonator transmission S 21 was measured with a network analyser as a function of the screening current I s and bias field B 0 . ( c ) The intrinsic quality factor of the resonator and the resonance frequency shift Δ f 0 = f 0 ( I s =0)− f 0 ( I s ) have been obtained from transmission curves of a , b (see Methods). Solid lines present polynomial fits. ( d ) The inductance L tot determines the resonance frequency according to , where C =20 pF and C c =2.2 pF. The inductance L tot =( L g + L k )/4+ L par contains contributions from loop inductance and parasitics, where L g =142 nH and L par = L g,par + L k0,par =40 nH with geometric inductances computed with a simulation software. The quadratic fit of d gives L k0 =147 nH and I *=34 mA for the kinetic inductance. Full size image The decrease in Cooper pair density n s with growing I s degrades the intrinsic quality factor Q i of the device ( Fig. 2c ) and enhances the resonator inductance L tot ( Fig. 2d ) due to the kinetic term given by equation (2), resulting in the resonance frequency shift Δ f 0 ( Fig. 2c ). The inductance change enables the derivation of parameters L k0 =147 nH and I *=34 mA. Assuming the nominal geometry of the superconducting strip ( l =80 mm, w =5 μm and h =165 nm), one can determine the penetration depth λ =1,100 nm for the NbN thin film. The value is somewhat larger than the zero-temperature magnetic penetration depth in the impure limit , where ħ = h /(2 π ) is the reduced Planck constant, ρ =750±90 μΩ cm the film resisitivity at room temperature and Δ=2.5 meV the gap energy at zero temperature for NbN [24] . Responsitivity To calculate magnetometer responsivity ∂ ε out /∂ B 0 , where ε out is the output voltage of the transmission measurement, we differentiate equations (1)–(3), , . At the resonance, the responsitivity can be approximated as where the resonator is excited with a voltage ε in and the total quality factor Q t = Q i Q ext /( Q i + Q ext ) along with the inductance L tot are functions of the bias current I s . The responsitivity given by equation (4) is valid from d.c. to a roll-off frequency f r ≈min{ f 0 /(2 Q t ), 1/(2 πτ r )}, where either the electric time constant of the resonator [25] or the quasiparticle recombination time τ r (ref. 26 ) restricts the device bandwidth. Ultimately, the device gain becomes limited by the excitation ε in generating an RF current (amplitude i L ) through inductance L tot . In the limit i L =2( I c − I s ), where the factor of two stems from the loop geometry, the magnetometer is driven to the normal state and the maximum gain for a given bias current I s becomes The measured device responsitivities G tot d |Im ε out |/ dB 0 and G tot d |Re ε out |/ dB 0 are depicted in Fig. 3a,b for quadrature ( Q ) and in-phase ( I ) components, respectively. The theoretical plots, using parameters derived from the transmission measurements, follow the measured data yielding G tot =490±30 V V −1 for the system gain, which is in reasonable agreement with the nominal value G nom =400 V V −1 . The large dynamic range of the detector is visualized with the aid of half-gain bandwidth, which converted to magnetic field gives Δ B 0 ≈600 nT. For a constant excitation ε in =6.3 mV, the current i L is a weak function of I s and can be approximated as i L ≈1.3 mA. In this case, flux trapping was observed below the resonance frequency f 0 ≈99.5 MHz corresponding to bias current of the order I s ≈9.2 mA, approximately fulfilling the maximum gain condition i L ~2( I c − I s ). 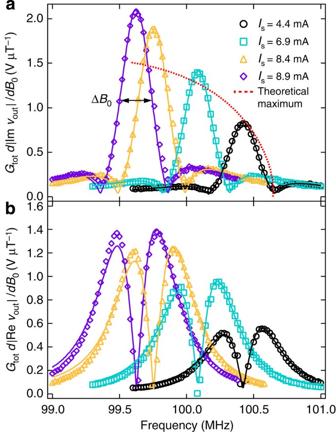Figure 3: Device gain. (a,b) The measured device responsitivitiesGtotd|Imεout|/dB0andGtotd|Reεout|/dB0representing quadrature and in-phase components, respectively, are shown along with theoretical fits (solid lines), where the total voltage gainGtotand bias currentIswere chosen as fitting parameters (see Methods). The total gainGtot=GLmixLattincludes the contributions from the amplificationG, mixer conversion lossLmixand other attenuationLattpresent in the setup. Ina, the equation (4) scaled withGtot=490±30 V V−1gives an estimate for theQ-component at resonance (red dashed line), in reasonable agreement with the measurements. The half-gain bandwidth for the largest peak expressed in terms of magnetic field is ΔB0≈600 nT. Figure 3: Device gain. ( a , b ) The measured device responsitivities G tot d |Im ε out |/ dB 0 and G tot d |Re ε out |/ dB 0 representing quadrature and in-phase components, respectively, are shown along with theoretical fits (solid lines), where the total voltage gain G tot and bias current I s were chosen as fitting parameters (see Methods). The total gain G tot = GL mix L att includes the contributions from the amplification G , mixer conversion loss L mix and other attenuation L att present in the setup. In a , the equation (4) scaled with G tot =490±30 V V −1 gives an estimate for the Q -component at resonance (red dashed line), in reasonable agreement with the measurements. The half-gain bandwidth for the largest peak expressed in terms of magnetic field is Δ B 0 ≈600 nT. Full size image Noise The fluctuation mechanisms peculiar to kinetic inductance devices are related to the dynamics of quasiparticle excitations: the thermal motion of the unpaired electrons and the stochastics of the quasiparticle density. The former, combined with the contribution from thermal fluctuations of the attenuated feeding line, generates Johnson voltage noise on resonance, where k B is the Boltzmann constant. Taking into account the coupling to the input of the amplifier and utilizing the equation (4), this can be mapped to magnetic field noise at the magnetometer loop The generation–recombination of the charge carriers, on the other hand, leads them to fluctuate according to spectral density S qp ( ω )=4 N qp τ r /(1+( ωτ r ) 2 ), where N qp = V n qp is the number of quasiparticles in the superconductor volume V . The field noise due to the generation–recombination process can be evaluated in the low-frequency limit f ≪ f r as (see Methods) where n qp is the density of quasiparticles. To study the noise properties, a device similar to the one characterized above was operated without external magnetic bias, using persistent current I s = m Φ 0 /( L g + L k ) with finite m to determine the operating point. The RF frequency and amplitude were set to approximately maximize the field responsitivity G tot dε out / dB 0 , and the experimental noise, shown in Fig. 4a , was recorded at high-gain operating point I s =7 mA. This is scaled to equivalent magnetic field noise in Fig. 4b . The white noise above 1 kHz corresponds to about 32±2 fT Hz −1/2 . The error limit stems from the uncertainty in mutual inductance M 1 calibration ( Fig. 1b ; see Methods). The peaks visible in the spectrum are mainly multiples of 50 Hz and interference located at low frequencies and from frequencies close to the carrier. 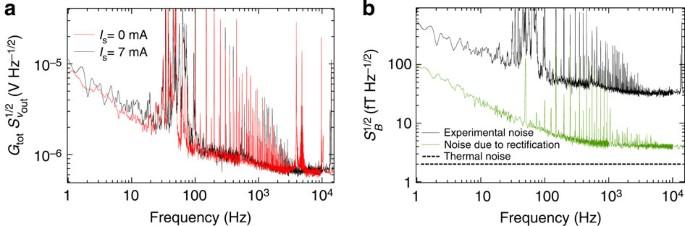Figure 4: Noise measurements. (a) The measured spectral density of the equivalent voltage noiseat high (Is=7 mA, black) as well as zero (Is=0 mA, red) field responsitivity. The measurement without the sensor yielded 540 nV Hz−1/2above 1 kHz and 2 μV Hz−1/2at 10 Hz (not shown here). (b) The magnetic field noiseforIs=7 mA (black), the field noisefrom rectification (equation (9), green) and theoretical sensor contribution dominated by the Johnson noise (dashed line). Figure 4: Noise measurements. ( a ) The measured spectral density of the equivalent voltage noise at high ( I s =7 mA, black) as well as zero ( I s =0 mA, red) field responsitivity. The measurement without the sensor yielded 540 nV Hz −1/2 above 1 kHz and 2 μV Hz −1/2 at 10 Hz (not shown here). ( b ) The magnetic field noise for I s =7 mA (black), the field noise from rectification (equation (9), green) and theoretical sensor contribution dominated by the Johnson noise (dashed line). Full size image To investigate the role of the electronics and any potential excess noise mechanisms, the noise spectrum was also recorded in a zero field-responsivity operating point I s =0 mA ( Fig. 4a ). Due to the similarity of the data at zero and finite field responsivity, we can exclude any noise mechanism related to random flux variations, such as the movement of trapped flux [27] or fluctuating spins of localized electrons on thin-film surfaces [28] , as the limiting factor in the experimental noise. Furthermore, we can also exclude the effect of parametric fluctuation of I *, since the inductance is to first order independent of I * at I s =0. After removing the sensor from the system, comparable noise values were measured for the setup, see Fig. 4 . We attribute the slight difference to stem from the difference in the impedance levels with respect to the amplifier noise optimum, as the source impedance on resonance is lower. A mechanism increasing the field noise at high-gain operating point is the RF amplitude fluctuations, manifesting itself through current rectification due to nonlinear inductance at high readout power, see Methods for details. The amplitude noise of the RF source was measured and an estimate of its (insignificant) contribution is shown in Fig. 4b . Using the device parameters and equations (6) and (7), we can calculate the theoretical noise floor of the sensor. The dominant contribution is the thermal noise . The contribution of generation–recombination noise is negligible as derived in the Methods. Therefore, after evaluating the magnitude of all the known noise processes, it is reasonable to conclude that the measured experimental noise is limited by the electronics. The geometry and the material of the kinetic inductance magnetometer correspond to those used in the pickup loops of SQUID magnetometers. Therefore, together with the results obtained from the noise measurements, low-frequency noise similar to that of SQUIDs can be anticipated. This should enable biomagnetic measurements at low frequencies, down to <1 Hz (magnetoencephalography or magnetocardiography) or in the range of ~kHz (ULF NMR and MRI). In comparison with SQUIDs, additional benefits include a high dynamic range, tolerance against ambient magnetic fields and immunity to RF interference. For the devices reported here, the dynamic range is several hundreds of nanotesla, outperforming typical SQUID magnetometers operated without feedback by two orders of magnitude. So far, the operation in Earth’s magnetic field has been verified, although the detailed characterization was done in shielded environment. The operability without shielding in higher ambient magnetic fields is expected, in contrast to SQUIDs for which the limiting factor is the magnetic penetration through the Josephson junction barrier, suppressing responsivity at fields of the order of Φ 0 /( λd ), where d is the dimension of the Josephson junction. The ambient field tolerance should be beneficial for techniques such as ULF MRI, where the recovery of the sensor after a relatively high magnetic field pulse is required. In planar unshielded SQUIDs, the large pulse typically suppresses the field responsivity as the magnetic flux trapped to superconductors couples to the junction [29] . Furthermore, unlike the SQUIDs [30] , the device should be insensitive to interference beyond f r , except in the narrow bandwidth of the resonator. General The experiments were performed in liquid helium using a cryoprobe equipped with two coaxial RF lines for the transmission measurement of the resonator as well as two d.c. lines for magnetic field generation. A magnetic shield made of Pb and cryoperm was mounted around the sample, resulting in ambient noise level below 5 fT Hz −1/2 in the white region measured with a SQUID magnetometer. Fabrication The NbN films were formed by reactive sputtering of niobium in nitrogen atmosphere on thermally oxidized silicon substrates. The devices were patterned through optical lithography and reactive-ion etching. The critical temperature and the resistivity of the film were verified by measuring the resistance as a function of temperature from reference structures on the same wafer as the magnetometers. Transmission measurements The field dependency of the device shown in Fig. 2 was characterized in transmission measurements. The bias field was varied by tuning the d.c. voltage supplied through resistors 2 R 1 =300 Ω and recording the corresponding transmission spectra with a network analyser. The spectra were then used for fitting the transmission S 21 =2 ε out / ε in =2 Z /(2 Z + Z 0 ) ( Fig. 1c ), where the complete impedance of the capacitively coupled resonator was employed. Capacitor values measured with an impedance analyser from similar test structures were assumed ( C c =2.2 pF and C =20 pF), while resonance frequency and quality factor were used as fitting parameters. The amplitude of the transmission was fixed to unity sufficiently far away from the resonance. The best fit was achieved with Z 0 =63 Ω. As a result, the curves of Fig. 2c were obtained. Solid lines represent polynomial fits containing all the necessary information for reproducing the transmission curves of Fig. 2a,b . Responsitivity measurements The device responsivities G tot dε out / dB 0 were measured with the setup of Fig. 5a . Two channels of an RF generator provide signals for excitation ε RF = ε 0,RF sin( ω RF t ) of the resonator and for a reference ε LO = ε 0,LO sin( ω LO t + φ ) of the mixer. The transmitted signal is amplified at room temperature with a low-noise amplifier and mixed down to d.c. ( ω LO = ω RF ). The d.c. signal is low-pass filtered, amplified and, finally, Fourier transformed to frequency domain. An attenuator (−40 dB) was placed at low temperature end of the input to reduce the noise originating from the room-temperature electronics and wiring. 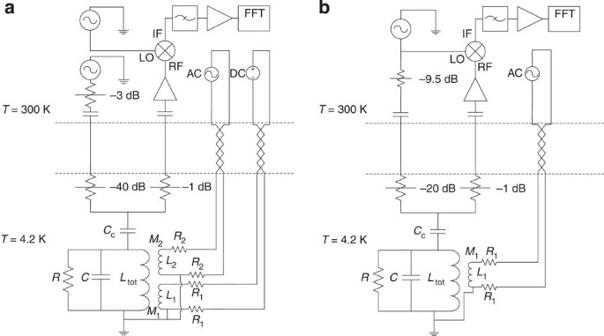Figure 5: Measurement setups. To eliminate the phase noise between LO and RF signals present in the responsitivity measurements (a), a single signal generator was adopted for the noise measurements (b). Figure 5: Measurement setups. To eliminate the phase noise between LO and RF signals present in the responsitivity measurements ( a ), a single signal generator was adopted for the noise measurements ( b ). Full size image The phase φ of the local oscillator (LO) was first manually tuned close to a value φ = φ max , where a maximum response (quadrature ( Q ) component) at a given resonance frequency f 0 is obtained. The responsitivity was also recorded at − π /2 offset giving the approximate in-phase ( I ) component. The IQ data were rotated in post processing to comply with the accurate value of φ max , yielding the plots in Fig. 3 . The root mean squared value of the carrier signal was set to 0.88 V corresponding to after the attenuators. Fitting was performed to measured data using functions of the form ( Q -component) and ( I -component) with G tot and I s selected as fitting parameters. Here transmission S 21 was computed using the fits of Fig. 2c and the total voltage gain G tot = GL mix L att includes contributions from the amplifiers G , mixer insertion loss L mix and other attenuation L att present in the setup. The bias current I s values for each plot are shown in the inset of Fig. 3a and the total gain G tot =490±30 V V −1 , which is close to the nominal gain G nom =400 V V −1 assuming G =62 dB, L mix =−8 dB and L att =−2 dB. Noise measurements For the noise measurements, the measurement setup was modified in the following ways ( Fig. 5b ). A nominally identical sample with slightly better responsitivity was adopted for the measurements. To remove the phase noise between the LO and the carrier, the two signals were obtained from a splitter supplied by a single RF voltage source. Furthermore, an adjustable attenuator was installed to room temperature to control the excitation voltage ε in . The device was operated in so-called persistent current mode, in which the magnetic flux m Φ 0 within the loop alone determines the operating point I s = m Φ 0 /( L g + L k ), eliminating the noise of the d.c. flux bias. A signal composed mainly of the Q -component was chosen for the measurement by using cables of proper length acting as a delay line. The device gain was set close to the maximum by biasing the device at the resonance frequency and adjusting the excitation voltage ε in to 12 mV. The voltage noise at the output was measured both for high ( I s =7 mA) and zero ( I s =0 mA) field responsitivity ( Fig. 4a ). The device gain was checked before and after the noise measurement yielding G tot dε out / dB 0 =20.3 V μT −1 . At our carrier frequency corresponding to the transmission minimum, the I -component responsivity is close to zero and the output is first-order insensitive to RF amplitude fluctuations. However, the inductance nonlinearity partially rectifies the RF excitation signal. In equation (2), the RF excitation current in the magnetometer loop can be contained by additional current term ( i L /2) sin( ωt ), where the factor of 1/2 stems from the fact that the current is divided into two branches. Thus, generalizing , replacing I s by in equation (2) and omitting extra RF terms, we get L k = L k0 (1+( I s / I *) 2 )+ L RF with L RF =( L k0 /8)( i L / I *) 2 . If there now exists RF amplitude fluctuation , it can be mapped to equivalent magnetic field noise , which is readily expressed as Now the relative fluctuation can be traced back to RF source, that is, . We measured this with the excitation level used in noise measurements and the result was converted to using equation (9) and i L ≈3 mA, see Fig. 4b . Calibration of mutual inductances Two printed circuit board (PCB) coils (inductances L 1 and L 2 ) were arranged around the sample to introduce magnetic bias and calibration fields. Mutual inductances M 1 and M 2 between the magnetometer and the off-chip coils were evaluated using the analytic formula of magnetic field around a straight wire of finite length where the current I flows from one end (point A) of the wire to the other (point B) and the magnetic field is calculated a distance r away from the wire (point C) defined by the angles θ 1 = ∠ (ABC) and θ 2 = ∠ (CAB). The model was found to reproduce the field profile measured with a magnetic field sensor (Alphalab Gaussmeter GM2) ~1 mm above the PCB, yielding M 1 =50±3 nH and M 2 =20±1.5 nH, where the error limits are related to the uncertainties in the position of the magnetometer. The calculated M 1 , combined with the derived inductances L g and L k0 , gives I c =10 mA for the magnetometer loop in line with the critical current measurements. Furthermore, the calibration of M 2 seems also accurate as discovered from responsitivity measurements with G tot ≈ G nom . Generation–recombination noise We derive the equivalent magnetic field noise S B ,gr stemming from the quasiparticle number fluctuation S N ( ω )=4 n qp Vτ r /(1+( ωτ r ) 2 ). The kinetic inductance can be estimated as L k ≈( n / n s ) L k0 =(1+ n qp / n s ) L k0 ≈(1+ N qp /( V n )) L k0 , where we approximate n s ≈ n , that is, a majority of the charge carriers is paired. The inductance fluctuation is derived as S L ( ω )=(∂ L /∂ N qp ) 2 S N ( ω )=( L k0 / V n s ) 2 S N ( ω ). Equation (7) follows now from S B ,gr ( ω )=(∂ L /∂ B 0 ) −2 S L ( ω ) assuming . Thus, the generation–recombination noise depends on parameters n s , n qp and τ r . As noted above, we assume that the paired carrier density n s approximately equals the total density n of electrons: n s ≈ n ~10 29 1 per m 3 (ref. 31 ). For our NbN films, the Cooper pair density is empirically found to follow relation n s /( n s + n qp )=1−( T / T c ) 2.5 (ref. 15 ). Using this combined with the relation of the intrinsic quality factor Q i = n s /( n qp ω 0 τ qp ), where τ qp is the quasiparticle thermalization time with a superconductor lattice, and the current dependency of Q i gives n qp / n s ≈0.1. The recombination time can be expressed as [26] where τ 0 is material-dependent electron–phonon interaction time and Δ is the energy gap of the superconductor. For NbN, an empirical relation τ 0 [s]=5 × 10 −10 T [K] −1.6 is typically found valid [32] leading to τ 0 ≈50 ps. The zero-temperature energy gap for NbN is Δ=2.5 meV (ref. 24 ). Although this is likely somewhat suppressed at the operating point, it will give a worst-case estimate for the noise. Finally, we get τ r ≈1.5 ns and using dL / dB 0 ≈3 mH T −1 at operating point. How to cite this article : Luomahaara, J. et al. Kinetic inductance magnetometer. Nat. Commun. 5:4872 doi: 10.1038/ncomms5872 (2014).